FAK transduces extracellular forces that orient the mitotic spindle and control tissue morphogenesis Spindle orientation is critical for proper morphogenesis of organs and tissues as well as for the maintenance of tissue morphology. Although significant progress has been made in understanding the mechanisms linking the cell cortex to the spindle and the well-documented role that extracellular forces play in spindle orientation, how such forces are transduced to the cortex remains poorly understood. Here we report that focal adhesion kinase (FAK) is necessary for correct spindle orientation and as a result, indispensable for proper epithelial morphogenesis in the vertebrate embryo. We show that FAK’s role in spindle orientation is dependent on its ability to localize at focal adhesions and its interaction with paxillin, but is kinase activity independent. Finally, we present evidence that FAK is required for external force-induced spindle reorientation, suggesting that FAK’s involvement in this process stems from a role in the transduction of external forces to the cell cortex. Defective spindle orientation is associated with developmental abnormalities often associated with severe diseases, including neurological disorders, polycystic kidneys and tumorigenesis [1] , [2] , [3] . Cortical pulling forces generated by dynein on astral microtubules define the position and orientation of the spindle. A conserved core protein complex composed of several proteins including LGN, NuMA and the G-protein subunit Gαi recruit dynein to the cortex. LGN localizes at the cell cortex of dividing cells and interacts with the plasma membrane-bound Gαi-GDP through its C-terminus and with NuMA (which binds to dynein directly) through its N-terminus [4] . Through different mechanisms the LGN/NuMA/Gαi complex localizes asymmetrically at the cortex, leading to determined localization of dynein [5] . Several factors have been shown to influence mitotic spindle orientation including cell polarity, cell shape and, more recently, external forces [6] , [7] . Fink et al. [7] , elegantly showed that external forces transmitted through the retraction fibres (RFs) can guide mitotic spindle orientation in adherent cells, whereas external forces have also been shown to control spindle orientation in vivo in the zebrafish EVL [8] . Despite an abundance of molecules identified as regulators of mitotic spindle positioning and orientation, including microtubule- and actin-associated proteins, kinases, cell polarity proteins, adherens junction proteins, transmembrane receptors and phosphoinositides [3] , [5] , [7] , [8] , [9] , [10] , [11] , [12] , [13] , [14] , [15] , how are external forces transmitted to the cell cortex and bias cortical cues is still poorly understood. The members of the focal adhesion (FA) complex are important mechanosensing molecules, and the FA complex itself can mature and change composition in response to external forces [16] . In this study, we explored the possibility that FAK, a major mechanosensing molecule regulated by mechanical forces, is involved in the regulation of spindle orientation [17] , [18] . We show that FAK is required for spindle orientation and that this function is related to FAK’s role in the transduction of mechanical signals from the extracellular environment to the cell. FAK is required for spindle orientation in adherent cells The fact that integrins have been shown to play a critical role in spindle orientation in several systems [15] , [19] coupled with the central role of FAK in the transduction of integrin signalling [20] , prompted us to investigate a possible role of FAK in spindle orientation. We begun by examining spindle orientation in FAK-null mouse embryonic fibroblasts (MEFs) and compared the results to those from FAK-nulls re-expressing WT-FAK. The mitotic spindle of adherent cells is normally parallel to the substratum [15] , so for each metaphase cell, thin optical sections were acquired along the Z axis and the angle between the two spindle poles with respect to the substrate was measured from Z reconstructions ( Fig. 1a,b ). The average spindle angle in FAK-null cells was 20.3±1.368° ( n =116), whereas this angle was 8.849±0.7483° ( n =95) in FAK re-expressing cells ( Fig. 1b,c ). In addition, 75% of the FAK-null cells showed a spindle angle greater than 10° compared with 32% in FAK re-expressing cells ( Fig. 1d ). Examination of spindle integrity and spindle centring revealed that loss of FAK does not affect spindle integrity or centring ( Supplementary Fig. 1a–e ) [15] . In addition, both electroporation of a previously characterized FAK morpholino (MO) [21] in Xenopus XL177 cells, as well as expression of a FAK dominant negative composed of the N and C termini of FAK (FF) [22] in NIH3T3 cells, lead to spindle misorientation confirming a requirement for FAK in spindle orientation ( Supplementary Fig. 1f–h ). 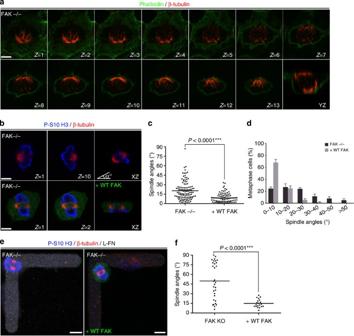Figure 1: FAK-null MEFs display spindle orientation defects. (a) Thin optical sections (0.37 μm) of a FAK-null metaphase cell and the correspondingYZ-projection image. (b) First and last optical sections from a Z-stack, showing the two spindle poles and theXZ-projection of a FAK-null metaphase cell and a FAK reconstituted cell (transfected with GFP FAK). (c) Scatter plots of the substrate to spindle angles (angleαshown inb) of FAK-null and WT-FAK reconstituted cells. The average spindle angle in FAK-null cells is 20.30±1.368° (n=116) and in WT-FAK reconstituted cells 8.849±0.7483° (n=95). Analysis of spindle orientation with a Mann–Whitney test showed statistically significant differences of the means of the spindle angles between the two samples, ***P<0.0001;n, number of metaphase cells, six independent experiments. (d) Quantification of the percentage of metaphase cells with substrate to spindle angles greater than 10°. 75% of FAK-null cells displayed spindle angles greater than 10° compared with 32% of FAK reconstituted cells. Error bands are s.e.m. (e) Representative images of FAK-null and FAK reconstituted metaphase cells on L-shaped fibronectin micropatterns. (f) Scatter plots ofXYspindle angles of FAK-null and WT-FAK reconstituted cells on L-shaped fibronectin micropatterns. The average spindle angle in FAK-null cells is 49.77±5.119° (n=31) and in WT-FAK reconstituted cells is 14.82±1.426° (n=20). Quantification of spindle orientation with a Mann–Whitney test showed statistically significant differences of the means of the spindle angles between the two samples, ***P<0.0001;n, number of metaphase cells, two independent experiments. Scale bars (a,b), 5 μm, (e) 10 μm. Figure 1: FAK-null MEFs display spindle orientation defects. ( a ) Thin optical sections (0.37 μm) of a FAK-null metaphase cell and the corresponding YZ -projection image. ( b ) First and last optical sections from a Z-stack, showing the two spindle poles and the XZ -projection of a FAK-null metaphase cell and a FAK reconstituted cell (transfected with GFP FAK). ( c ) Scatter plots of the substrate to spindle angles (angle α shown in b ) of FAK-null and WT-FAK reconstituted cells. The average spindle angle in FAK-null cells is 20.30±1.368° ( n =116) and in WT-FAK reconstituted cells 8.849±0.7483° ( n =95). Analysis of spindle orientation with a Mann–Whitney test showed statistically significant differences of the means of the spindle angles between the two samples, *** P <0.0001; n , number of metaphase cells, six independent experiments. ( d ) Quantification of the percentage of metaphase cells with substrate to spindle angles greater than 10°. 75% of FAK-null cells displayed spindle angles greater than 10° compared with 32% of FAK reconstituted cells. Error bands are s.e.m. ( e ) Representative images of FAK-null and FAK reconstituted metaphase cells on L-shaped fibronectin micropatterns. ( f ) Scatter plots of XY spindle angles of FAK-null and WT-FAK reconstituted cells on L-shaped fibronectin micropatterns. The average spindle angle in FAK-null cells is 49.77±5.119° ( n =31) and in WT-FAK reconstituted cells is 14.82±1.426° ( n =20). Quantification of spindle orientation with a Mann–Whitney test showed statistically significant differences of the means of the spindle angles between the two samples, *** P <0.0001; n , number of metaphase cells, two independent experiments. Scale bars ( a , b ), 5 μm, ( e ) 10 μm. Full size image The mitotic spindle of adherent cells is normally parallel to the substratum, whereas it is oriented through mechanical forces exerted by RFs in the XY [23] . It is thus possible to force the spindle of adherent cells into a defined orientation by plating cells onto micropatterned surfaces. To determine whether loss of FAK affects XY spindle orientation, we used L-shaped fibronectin micropatterns. The mitotic spindle of cells grown on this pattern is normally parallel to the hypotenuse of the triangle formed by the L [23] . Examination of spindle orientation on L-shaped microprints revealed loss of spindle orientation of FAK-null cells in the XY plane. Specifically, under these conditions, FAK-null cells display randomized spindles with an average angle of deviation of 49.77±5.119° ( n =31), compared with 14.82±1.426° ( n =20) in FAK reconstituted cells ( Fig. 1e,f ). These results show that FAK is required both for spindle alignment with the substrate as well as for force-dependent orientation associated with RFs. As both cell shape and forces have been shown to influence spindle orientation [6] , [7] , [8] , we also quantified spindle orientation on bar-shaped patterns, which generate greater cell shape anisotropy. FAK-nulls on such patterns display a moderate but statistically significant reduction of misorientation compared with cells on L-shapes, suggesting that the primary defect on FAK-nulls is in force-dependent orientation ( Supplementary Fig. 1i ). Spindle orientation is determined by the ECM distribution Integrin-based cell adhesion to extracellular matrix (ECM) components orients the mitotic spindle of cultured cells parallel to the plane of the substrate [15] . Although the mechanism through which this Z axis orientation is accomplished is sometimes assumed to be the same as in the case of orientation in the XY plane, this has never been addressed directly [24] , [25] . The fact that FAK-null cells fail to orient their spindle both in response to micropatterns as well as with respect to the plane of the substrate suggests that the two orientation processes share a common mechanism. It is likely that the absence of RFs at the basal and apical areas of a spherical mitotic cell would automatically lead to the exclusion of a vertical division with respect to the substrate, as no force is applied in that direction. In order to address this possibility, we exposed cells to two parallel substrate planes by sandwiching them between coverslips. After cells attached to the first coverslip, a second was positioned over them using silicone grease bridges to hold it in place ( Fig. 2a ). As shown, HeLa cells primarily adhere and spread on the bottom coverslip while maintaining a small area in contact with the top coverslip ( Fig. 2a,b ). Once they round up, the majority of RFs are formed on the bottom coverslip, however, RFs also form at the top ( Fig. 2a,b ). Cells under these conditions fail to orient their spindles parallel to the substrate and often divide completely perpendicular to the substratum ( Fig. 2b–d ). This suggests that RFs under these conditions apply forces perpendicular to the substrate plane leading to the change in spindle orientation. In order to ensure that spindle reorientation is a result of integrin-dependent adhesion, we repeated the experiment using fibronectin bottom coverslips and poly- L -lysine (PLL) coverslips on top ( Fig. 2a ). In agreement with previous work, spindles under these conditions remain parallel to the substratum ( Fig. 2c,d ), indicating that integrin-based adhesions are required to elicit spindle orientation changes [15] . Overall, these results suggest that the mechanism for spindle orientation in the XY and Z axis is common and depends on the spatial distribution of the ECM, which defines the distribution of RFs and subsequently, the spatial distribution of forces applied on the cell cortex. 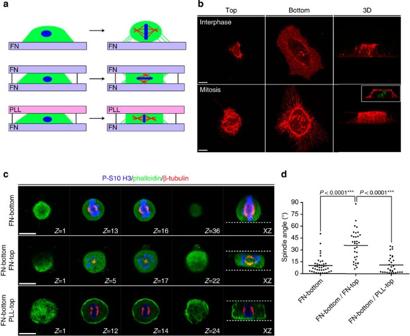Figure 2: The mechanism of spindle orientation in theXYandZaxis is common and depends on the spatial distribution of the retraction fibres. (a) Schematic representation of the experimental setup to determine the role of RFs inZaxis spindle orientation: cells seeded on a fibronectin (FN)-coated coverslip, sandwiched between two FN-coated coverslips or sandwiched between a FN-coated coverslip and a PLL-coated coverslip and imaged during cell division. (b) Confocal images of live memCherry-transfected HeLa cells confined between two FN-coated coverslips. Optical sections showing the top and the bottom of an interphase cell and a three-dimensional (3D) reconstruction show how the cell adheres on both coverslips. In the lower panel, optical sections of the top and the bottom of a mitotic cell and a 3D reconstruction show the distribution of the RFs. The small rectangle in the 3D reconstruction of the lower panel shows a side view of the mitotic cell where the metaphase plate (green) is not perpendicular to the substrate. (c)Z-stacks (0.37 μm interval) and the correspondingXZside view of representative mitotic cells grown under the experimental settings shown ina. Cells were fixed and stained for actin, β-tubulin and P-S10 H3. The white dashed lines represent the coverslips. (d) Scatter plots of spindle angles relative to the substrate of the cells grown under the three conditions. The average spindle angle for cells grown in two-dimensional is 10.17±1.699° (n=39), in cells grown between two FN-coated coverslips 35.72±3.405° (n=33) and in cells grown between a FN-coated and a PLL-coated coverslip 11.01±1.987° (n=31). Quantification of spindle orientation with a Mann–Whitney test shows statistically significant differences of the means of the spindle angles between the indicated samples, ***P<0.0001;n, number of metaphase cells, three independent experiments. Scale bars (b,c), 10 μm. Figure 2: The mechanism of spindle orientation in the XY and Z axis is common and depends on the spatial distribution of the retraction fibres. ( a ) Schematic representation of the experimental setup to determine the role of RFs in Z axis spindle orientation: cells seeded on a fibronectin (FN)-coated coverslip, sandwiched between two FN-coated coverslips or sandwiched between a FN-coated coverslip and a PLL-coated coverslip and imaged during cell division. ( b ) Confocal images of live memCherry-transfected HeLa cells confined between two FN-coated coverslips. Optical sections showing the top and the bottom of an interphase cell and a three-dimensional (3D) reconstruction show how the cell adheres on both coverslips. In the lower panel, optical sections of the top and the bottom of a mitotic cell and a 3D reconstruction show the distribution of the RFs. The small rectangle in the 3D reconstruction of the lower panel shows a side view of the mitotic cell where the metaphase plate (green) is not perpendicular to the substrate. ( c ) Z -stacks (0.37 μm interval) and the corresponding XZ side view of representative mitotic cells grown under the experimental settings shown in a . Cells were fixed and stained for actin, β-tubulin and P-S10 H3. The white dashed lines represent the coverslips. ( d ) Scatter plots of spindle angles relative to the substrate of the cells grown under the three conditions. The average spindle angle for cells grown in two-dimensional is 10.17±1.699° ( n =39), in cells grown between two FN-coated coverslips 35.72±3.405° ( n =33) and in cells grown between a FN-coated and a PLL-coated coverslip 11.01±1.987° ( n =31). Quantification of spindle orientation with a Mann–Whitney test shows statistically significant differences of the means of the spindle angles between the indicated samples, *** P <0.0001; n , number of metaphase cells, three independent experiments. Scale bars ( b , c ), 10 μm. Full size image FAK’s kinase activity is dispensable for spindle orientation One of the central mechanisms through which FAK transduces integrin signals and controls FA turnover is through phosphorylation of downstream targets [26] . We thus examined if FAK’s kinase activity is important in spindle orientation both in the Z axis and in the XY plane by transfecting FAK-null cells with the kinase-inactive mutant FAK-K454R [27] . The results from these experiments are nearly identical to those for WT-FAK suggesting that FAK’s kinase activity is dispensable for correct spindle orientation ( Fig. 3a,d ). Due to the unexpected nature of this result we went on to confirm it using the FAK kinase inhibitor PF-228 in HeLa and NIH3T3 cells [28] . Both cell lines were treated with the inhibitor for 24 h and inhibitor effectiveness was evaluated by western blotting ( Supplementary Fig. 2c,f ). Quantification of spindle angles in inhibitor treated cells confirmed that inhibition of FAK’s kinase activity does not affect spindle orientation, confirming that spindle orientation does not require FAK’s enzymatic activity ( Supplementary Fig. 2a,b and d,e ). 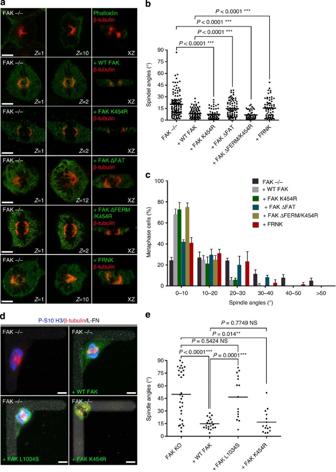Figure 3: The FAK kinase and FAT domains, but not the kinase activity, are required for correct spindle orientation. (a) First and last optical sections fromZ-stacks and the correspondingXZ-projections of a FAK-null metaphase cell and FAK-nulls transfected with WT-FAK, FAK-K454R, FAKΔFAT, ΔFERM/K454R and FRNK. (b) Scatter plots of substrate to spindle angles from nulls and cells transfected with the constructs ina. The average spindle angle in FAK-nulls transfected with FAK-K454R is 7.200±0.8812° (n=58), FAKΔFAT 15.08±1.333° (n=61), ΔFERM/K454R 6.586±0.7927° (n=48) and FRNK 15.37±1.478° (n=63). A Kruskal–Wallis test gave statistically significant results (***P<0.0001) indicating that at least one of the sample distributions is different from the other samples. Analysis with Mann–Whitney tests showed statistically significant differences of the means of the spindle angles for the indicated samples, ***P<0.0001;n, number of metaphase cells, three independent experiments. Comparison between WT-FAK and FAK-K454R, WT-FAK and ΔFERM/K454R, FAK−/− and FAKΔFAT, and FAK−/− and FRNK with Mann–Whitney tests revealed that the differences in the average spindle angles are statistically insignificant (not significant (NS):P=0.1713, NS:P=0.1627, NS:P=0.6755 and NS:P=0.6455, respectively). (c) Plots (means±s.e.m.) showing the percentage of cells that displayed spindle angles greater than 10°, which were 27%, 58%, 25% and 59% for the FAK-nulls transfected with FAK-K454R, FAKΔFAT, ΔFERM/K454R and FRNK, respectively. (d) Representative images of FAK-null, and FAK-nulls transfected with the WT-FAK, FAK-L1034S or FAK-K454R constructs on L-shaped fibronectin micropatterns. (e) Scatter plots ofXYspindle angles of the samples ind. The average spindle angle in FAK-L1034S-transfected cells is 46.61±6.538° (n=15) and in FAK-K454R 17.82±4.912° (n=10). Statistical analysis with Mann–Whitney tests showed statistically significant differences of the means of the spindle angles between FAK-null- and FAK-K454R-expressing cells (**P=0.014) and between FAK re-expressing cells and FAK-L1034S-expressing cells (***P<0.0001), but no statistically significant differences between FAK-null- and FAK-L1034S-expressing cells (NS:P=0.5424) or between WT-FAK- and FAK-K454R-expressing cells (NS:P=0.7749);n, number of metaphase cells, two independent experiments. Scale bars (a), 5 μm, (d) 10 μm. Figure 3: The FAK kinase and FAT domains, but not the kinase activity, are required for correct spindle orientation. ( a ) First and last optical sections from Z -stacks and the corresponding XZ -projections of a FAK-null metaphase cell and FAK-nulls transfected with WT-FAK, FAK-K454R, FAKΔFAT, ΔFERM/K454R and FRNK. ( b ) Scatter plots of substrate to spindle angles from nulls and cells transfected with the constructs in a . The average spindle angle in FAK-nulls transfected with FAK-K454R is 7.200±0.8812° ( n =58), FAKΔFAT 15.08±1.333° ( n =61), ΔFERM/K454R 6.586±0.7927° ( n =48) and FRNK 15.37±1.478° ( n =63). A Kruskal–Wallis test gave statistically significant results (*** P <0.0001) indicating that at least one of the sample distributions is different from the other samples. Analysis with Mann–Whitney tests showed statistically significant differences of the means of the spindle angles for the indicated samples, *** P <0.0001; n , number of metaphase cells, three independent experiments. Comparison between WT-FAK and FAK-K454R, WT-FAK and ΔFERM/K454R, FAK−/− and FAKΔFAT, and FAK−/− and FRNK with Mann–Whitney tests revealed that the differences in the average spindle angles are statistically insignificant (not significant (NS): P =0.1713, NS: P =0.1627, NS: P =0.6755 and NS: P =0.6455, respectively). ( c ) Plots (means±s.e.m.) showing the percentage of cells that displayed spindle angles greater than 10°, which were 27%, 58%, 25% and 59% for the FAK-nulls transfected with FAK-K454R, FAKΔFAT, ΔFERM/K454R and FRNK, respectively. ( d ) Representative images of FAK-null, and FAK-nulls transfected with the WT-FAK, FAK-L1034S or FAK-K454R constructs on L-shaped fibronectin micropatterns. ( e ) Scatter plots of XY spindle angles of the samples in d . The average spindle angle in FAK-L1034S-transfected cells is 46.61±6.538° ( n =15) and in FAK-K454R 17.82±4.912° ( n =10). Statistical analysis with Mann–Whitney tests showed statistically significant differences of the means of the spindle angles between FAK-null- and FAK-K454R-expressing cells (** P =0.014) and between FAK re-expressing cells and FAK-L1034S-expressing cells (*** P <0.0001), but no statistically significant differences between FAK-null- and FAK-L1034S-expressing cells (NS: P =0.5424) or between WT-FAK- and FAK-K454R-expressing cells (NS: P =0.7749); n , number of metaphase cells, two independent experiments. Scale bars ( a ), 5 μm, ( d ) 10 μm. Full size image The kinase and FAT domains are vital for spindle orientation The above results suggest that FAK’s function in spindle orientation is a scaffolding one. Given the previously identified role of integrins in spindle orientation, we postulated that FA localization of FAK would be necessary for its function in this context. The FAT domain is both necessary and sufficient for FAK’s FA localization [29] . Expression of a FAKΔFAT mutant in FAK nulls failed to rescue spindle orientation defects, suggesting that the FAT domain and FA localization are important ( Fig. 3a–c ). In agreement with this, we observed that although most FA complexes disassemble in mitotic cells, small FAK-positive adhesive complexes are retained along the RFs at areas where the fibres contact the ECM ( Supplementary Fig. 3a,b ). This suggests that FAK may be regulating spindle orientation by facilitating the transduction of external forces, generated at the ECM–RF interface, to the cell cortex, a notion supported by the fact that FAK-null MEFs do form RFs ( Supplementary Fig. 3a ). We went on to examine a possible role of the FERM (4.1 protein, ezrin, radixin, moesin) domain, which has been shown to interact with several proteins involved in spindle orientation, such as the Arp2/3 complex and integrins [30] , [31] . FAK-nulls were transfected with a kinase-dead mutant of FAK that lacks the FERM domain (ΔFERM/K454R). As shown, expression of ΔFERM/K454R rescued the phenotype of spindle misorientation with the same efficiency as WT-FAK and FAK-K454R, suggesting that the FERM domain is dispensable ( Fig. 3a–c ). Given the fact that the kinase activity and the FERM domain are both dispensable, we went on to express the C-terminal non-catalytic part of the protein referred to as FAK-related non-kinase (FRNK) [32] . FRNK failed to rescue spindle orientation indicating that the FAT-containing C-terminus is not sufficient ( Fig. 3a–c ). This result suggests that despite the fact that the kinase activity is not necessary for correct spindle orientation, the kinase domain itself is revealing a novel kinase domain dependent but kinase activity-independent function. A FAK paxillin interaction is critical for spindle orientation In order to probe the role of the FAT domain further, we expressed variants of FAK with point mutations that abolish interactions with known FAK-binding partners. The FAK C-terminus has been shown to be necessary for interactions with several proteins including talin, paxillin, RhoGEF and Grb2 (refs 33 , 34 , 35 , 36 ). Specifically, several lines of evidence suggest that the interactions with paxillin and talin are important for FAK’s localization at FAs. We thus initially used two previously characterized point mutants FAK-E1015A and FAK-L1034S, which have been shown to abolish the interaction of FAK with talin and paxillin, respectively, whereas retaining FA localization [35] , [37] . As shown, expression of the FAK-E1015A mutant can effectively rescue orientation defects indicating that the FAK–talin interaction is not necessary ( Fig. 4a,b ). However, expression of the FAK-L1034S point mutant failed to rescue spindle orientation defects both in the Z axis and in the XY plane ( Figs 3d,e and 4a,b ). As the L1034S mutation has recently been shown to affect the structure of the four helix bundle that makes up the FAT domain and in addition, leads to loss of the FAK–RhoGEF interaction [33] , [38] , we confirmed this result using the FAK-I936E/I998E mutant that specifically abolishes paxillin binding without affecting structure [38] ( Fig. 4a,b ). These results suggest that FA localization is not sufficient for FAK’s function in spindle orientation and requires the interaction with paxillin, which similar to FAK, also localizes at RFs ( Supplementary Fig. 3b ). 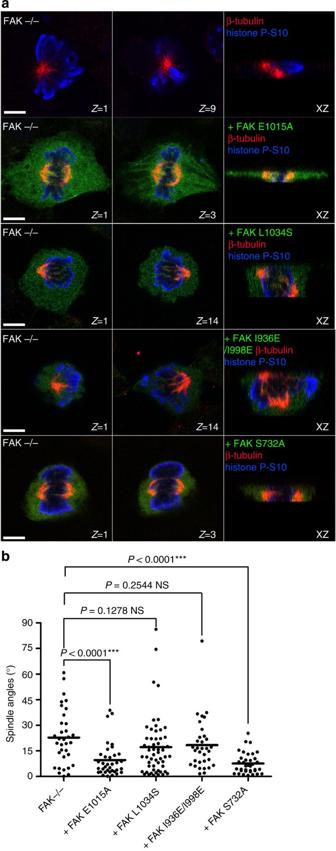Figure 4: FAK–paxillin interaction is necessary for proper spindle orientation in adherent cells. (a) Optical sections fromZ-stacks, showing the position of each spindle pole and theXZ-projections from a FAK-null metaphase cell and FAK-nulls transfected with the indicated mutants. (b) Scatter plots of measured substrate to spindle angles for FAK-nulls and FAK-nulls transfected with the indicated mutants. The average spindle angle in FAK-nulls is 22.77±2.780° (n=34), in FAK-null cells transfected with FAK-E1015A is 9.527±1.651° (n=36), in FAK-null cells transfected with FAK-L1034S is 17.14±2.303° (n=56), in FAK-null cells transfected with FAK-I936E/I998E is 18.37±2.624° (n=33) and in FAK-nulls transfected with FAK-S732A is 7.542±1.021° (n=36). Quantification of spindle orientation with a Mann–-Whitney test showed statistically significant differences of the means of the spindle angles between FAK-null and FAK-E1015A (***P<0.0001) and FAK-null and FAK-S732A (***P<0.0001) but not statistically significant differences between FAK-null and FAK-L1034S (not significant (NS):P=0.1278) and between FAK-null- and FAK-I936E/I998E-expressing cells (NS:P=0.2544);n, number of metaphase cells, two independent experiments. Scale bars (a), 5 μm. Figure 4: FAK–paxillin interaction is necessary for proper spindle orientation in adherent cells. ( a ) Optical sections from Z -stacks, showing the position of each spindle pole and the XZ -projections from a FAK-null metaphase cell and FAK-nulls transfected with the indicated mutants. ( b ) Scatter plots of measured substrate to spindle angles for FAK-nulls and FAK-nulls transfected with the indicated mutants. The average spindle angle in FAK-nulls is 22.77±2.780° ( n =34), in FAK-null cells transfected with FAK-E1015A is 9.527±1.651° ( n =36), in FAK-null cells transfected with FAK-L1034S is 17.14±2.303° ( n =56), in FAK-null cells transfected with FAK-I936E/I998E is 18.37±2.624° ( n =33) and in FAK-nulls transfected with FAK-S732A is 7.542±1.021° ( n =36). Quantification of spindle orientation with a Mann–-Whitney test showed statistically significant differences of the means of the spindle angles between FAK-null and FAK-E1015A (*** P <0.0001) and FAK-null and FAK-S732A (*** P <0.0001) but not statistically significant differences between FAK-null and FAK-L1034S (not significant (NS): P =0.1278) and between FAK-null- and FAK-I936E/I998E-expressing cells (NS: P =0.2544); n , number of metaphase cells, two independent experiments. Scale bars ( a ), 5 μm. Full size image Several reports revealed a role for FAK at centrosomes and basal bodies [39] , [40] , [41] . Deletion of FAK has been shown to lead to defective ciliogenesis, increases in centrosome numbers, defects in microtubule organization and nuclear movement as well as multipolar and disorganized spindles [39] , [41] . We wanted to examine if spindle misorientation in FAK nulls was related to the centrosomal functions of FAK and took advantage of the central role that phosphorylation of S732 by Cdk5 has in this context [41] . Expression of the S732A mutant effectively rescued spindle misorientation, suggesting that phosphorylation of this residue by Cdk5 is not important for FAK’s function in spindle orientation ( Fig. 4a,b ). FAK’s role in spindle orientation is conserved in the embryo Mechanisms controlling spindle orientation have been shown to be conserved between adherent cells and the in vivo setting [4] , [24] . Spindle orientation has been studied extensively especially in epithelia as oriented cell divisions are critical to several aspects of embryonic morphogenesis. We went on to examine a possible involvement of FAK in spindle orientation of epithelial tissues. The outer epithelium of Xenopus provides a good model as its well documented that cell divisions in this tissue are parallel to the plane of the epithelium [42] , [43] . Indirect immunofluorecence using FAK- and paxillin-specific antibodies revealed that both FAK and paxillin localize at the cell cortex and are enriched at the apical region of these cells ( Supplementary Fig. 4a,b ). We microinjected 50 ng of a previously characterized FAK MO [21] , [40] , [44] at the one-cell stage and imaged cell divisions of the outermost epithelial layer at early neurula. As shown, FAK knockdown (confirmed by western blot, Supplementary Fig. 5b ) leads to spindle orientation defects in intact embryos, whereas expression of the FAK dominant-negative FF [22] also induces spindle misorientation ( Supplementary Fig. 5a ). In order to facilitate imaging and quantification, further analysis was carried out in dissected animal caps (ACs) from morphant control and rescued embryos. As shown, both the FAK MO as well as expression of FF lead to loss of spindle orientation, whereas expression of WT-FAK effectively rescued the phenotype ( Fig. 5a–c and Supplementary Fig. 5d,e ). Staining with the tight junction marker ZO-1 revealed that apicobasal polarity is not affected in FAK morphants, whereas other polarized molecules involved in spindle orientation like the Par6/3-aPKC complex also remain properly localized even in cells with completely misoriented spindles [45] , [46] ( Supplementary Fig. 6a–c ). We went on to examine if LGN cortical enrichment was affected, however, as shown, LGN is localized at the cell cortex and is enriched at the areas across the spindle in both control and FAK morphant cells ( Supplementary Fig. 6d,e ). Despite the fact that the spindle is misoriented in FAK morphants, LGN is clearly enriched at the spindle capture regions, suggesting that FAK is not required for spindle capture but for the correct localization of the NuMA, LGN and Gαi-GDP complex responsible for astral microtubule capture and spindle orientation. 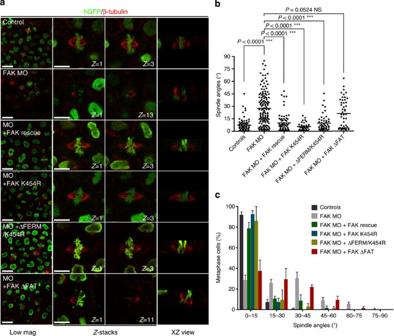Figure 5: FAK is necessary for spindle orientation in theXenopusepithelium and displays similar functional determinants as in adherent cells. (a) Low-magnification images of theXenopusouter epithelium showing mitotic cells (first column), optical sections showing each spindle pole (second, third column) andXZ-projections from representative metaphase cells of control, morphant and embryos rescued with indicated FAK mutants.Xenopusepithelia were stained with β-tubulin and anti-GFP antibodies. (b) Scatter plots of the spindle to plane of the epithelium angles from embryos shown ina. The average angle in control cells is 7.343±0.9881° (n=67), in FAK morphants is 27.50±1.682° (n=142), in cells rescued with the FAK-Rescue construct is 10.09±1.429° (n=64), in cells rescued with the FAK-K454R construct is 5.617±0.7739° (n=36), in cells rescued with the ΔFERM/K454R construct is 9.700±1.377° (n=50) and in FAK MO epithelial co-injected with the FAKΔFAT construct is 21.03±2.530° (n=48). A Kruskal–Wallis test gave statistically significant results (***P<0.0001). Analysis with Mann–Whitney tests showed statistically significant differences of the means of the spindle angles between the indicated samples, ***P<0.0001;n, number of metaphase cells, three independent experiments. Comparison between FAK-Rescue and FAK-K454R, FAK-Rescue and ΔFERM/K454R, FAK MO and FAKΔFAT with Mann–Whitney tests showed statistically insignificant differences of the means of the spindle angles (not significant (NS):P=0.1343, NS:P=0.6498 and NS:P=0.0524, respectively). (c) Plots (means±s.e.m) showing the percentage of metaphase cells with spindle to plane of the epithelium angles greater than 15°. These were 8%, 71%, 21%, 8%, 14% and 62.5% for control, FAK MO, FAK MO+FAK-Rescue, FAK MO+FAK-K454R, FAK MO+ΔFERM/K454R and FAK MO+FAKΔFAT, respectively. Scale bars: (a) low magnification: 20 μm, high magnification: 10 μm. Figure 5: FAK is necessary for spindle orientation in the Xenopus epithelium and displays similar functional determinants as in adherent cells. ( a ) Low-magnification images of the Xenopus outer epithelium showing mitotic cells (first column), optical sections showing each spindle pole (second, third column) and XZ -projections from representative metaphase cells of control, morphant and embryos rescued with indicated FAK mutants. Xenopus epithelia were stained with β-tubulin and anti-GFP antibodies. ( b ) Scatter plots of the spindle to plane of the epithelium angles from embryos shown in a . The average angle in control cells is 7.343±0.9881° ( n =67), in FAK morphants is 27.50±1.682° ( n =142), in cells rescued with the FAK-Rescue construct is 10.09±1.429° ( n =64), in cells rescued with the FAK-K454R construct is 5.617±0.7739° ( n =36), in cells rescued with the ΔFERM/K454R construct is 9.700±1.377° ( n =50) and in FAK MO epithelial co-injected with the FAKΔFAT construct is 21.03±2.530° ( n =48). A Kruskal–Wallis test gave statistically significant results (*** P <0.0001). Analysis with Mann–Whitney tests showed statistically significant differences of the means of the spindle angles between the indicated samples, *** P <0.0001; n , number of metaphase cells, three independent experiments. Comparison between FAK-Rescue and FAK-K454R, FAK-Rescue and ΔFERM/K454R, FAK MO and FAKΔFAT with Mann–Whitney tests showed statistically insignificant differences of the means of the spindle angles (not significant (NS): P =0.1343, NS: P =0.6498 and NS: P =0.0524, respectively). ( c ) Plots (means±s.e.m) showing the percentage of metaphase cells with spindle to plane of the epithelium angles greater than 15°. These were 8%, 71%, 21%, 8%, 14% and 62.5% for control, FAK MO, FAK MO+FAK-Rescue, FAK MO+FAK-K454R, FAK MO+ΔFERM/K454R and FAK MO+FAKΔFAT, respectively. Scale bars: ( a ) low magnification: 20 μm, high magnification: 10 μm. Full size image We went on to examine if the functional requirements revealed from experiments in FAK-null MEFs were conserved in the embryo. FAK MO was co-injected with mutants of FAK as shown in Fig. 5a . These results show that both the kinase activity and the FERM domain are dispensable, whereas the kinase and FAT domains are essential for correct spindle orientation in the epithelium ( Fig. 5a–c ). In addition, a paxillin-binding mutant failed to rescue spindle orientation defects ( Fig. 6a,b ), whereas use of a paxillin MO [47] (paxillin downregulation was confirmed by western blot, Supplementary Fig. 5c ) elicited spindle orientation defects. These defects were rescued by the expression of a Paxillin-Rescue construct ( Fig. 6c,d ), suggesting that the paxillin–FAK interaction is also critical, for FAK’s function in this process, in vivo [47] . Overall, these results suggest that FAK’s role in spindle orientation is conserved in the embryo. 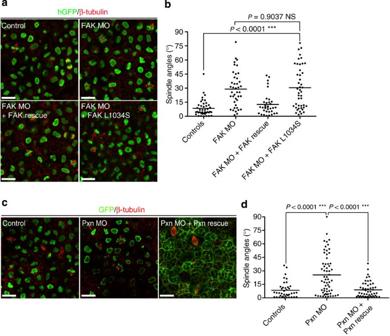Figure 6: The FAK–Paxillin interaction is necessary for spindle orientation ofXenopusepithelial cells. (a) Confocal images of epithelial cells from a control embryo, an embryo injected with FAK MO alone, FAK MO+FAK-Rescue and FAK MO+FAK-L1034S. HistoneGFP was used as a linage tracer and embryos were stained for β-tubulin and GFP. (b) Scatter plots of spindle to plane of the epithelium angles. The average angle in control cells is 8.462±1.324° (n=42), in FAK morphants is 28.88±2.909° (n=41), in rescued cells is 12.57±1.980° (n=35) and in FAK MO+FAK-L1034S-injected cells is 30.42±3.372° (n=45). Statistical analysis with a Mann–Whitney test showed statistically significant differences of the means of the spindle angles between control and FAK MO+FAK-L1034S (***P<0.0001) but no statistically significant differences between FAK morphants and FAK MO+FAK-L1034S-injected embryos (not significant (NS):P=0.9037);n, number of metaphase cells, two independent experiments. (c)Xenopusepithelium of a control embryo injected with histoneGFP, Pxn MO (100 ng Pxn MO+histoneGFP) and Pxn MO+Pxn-Rescue construct.Xenopusepithelia were stained for β-tubulin and GFP. (d) Scatter plots of spindle to plane of the epithelium angles. The average spindle angle in control cells is 8.282±1.433° (n=40), in Paxillin morphants is 25.37±2.774° (n=62) and in rescued cells is 8.761±1.226° (n=51). Statistical analysis with a Mann–Whitney test shows statistically significant differences of the means of the spindle angles between the indicated samples, ***P<0.0001;n, number of metaphase cells, two independent experiments. Scale bars (a,c), 20 μm. Figure 6: The FAK–Paxillin interaction is necessary for spindle orientation of Xenopus epithelial cells. ( a ) Confocal images of epithelial cells from a control embryo, an embryo injected with FAK MO alone, FAK MO+FAK-Rescue and FAK MO+FAK-L1034S. HistoneGFP was used as a linage tracer and embryos were stained for β-tubulin and GFP. ( b ) Scatter plots of spindle to plane of the epithelium angles. The average angle in control cells is 8.462±1.324° ( n =42), in FAK morphants is 28.88±2.909° ( n =41), in rescued cells is 12.57±1.980° ( n =35) and in FAK MO+FAK-L1034S-injected cells is 30.42±3.372° ( n =45). Statistical analysis with a Mann–Whitney test showed statistically significant differences of the means of the spindle angles between control and FAK MO+FAK-L1034S (*** P <0.0001) but no statistically significant differences between FAK morphants and FAK MO+FAK-L1034S-injected embryos (not significant (NS): P =0.9037); n , number of metaphase cells, two independent experiments. ( c ) Xenopus epithelium of a control embryo injected with histoneGFP, Pxn MO (100 ng Pxn MO+histoneGFP) and Pxn MO+Pxn-Rescue construct. Xenopus epithelia were stained for β-tubulin and GFP. ( d ) Scatter plots of spindle to plane of the epithelium angles. The average spindle angle in control cells is 8.282±1.433° ( n =40), in Paxillin morphants is 25.37±2.774° ( n =62) and in rescued cells is 8.761±1.226° ( n =51). Statistical analysis with a Mann–Whitney test shows statistically significant differences of the means of the spindle angles between the indicated samples, *** P <0.0001; n , number of metaphase cells, two independent experiments. Scale bars ( a , c ), 20 μm. Full size image FAK transduces external forces to the spindle Recent work has revealed that external forces can induce mitotic spindle rotation in adherent mammalian cells [7] , [25] , whereas cells of the EVL in zebrafish orient their mitotic spindle preferentially along the main axis of tension-promoting tissue spreading during epiboly [8] . To determine if external forces can induce spindle rotation in Xenopus, we placed mid-gastrula embryos in silicone-chambered slides and imaged them live under conditions where the embryo was being slightly depressed exerting mechanical force on the epithelium and in the absence of external force. As shown, under mechanical stimulation, the average spindle rotation increased by 50% and the same was true with respect to the frequency of rotation ( Fig. 7a–c ). These results show that application of external force can induce spindle rotation in vivo in a similar manner to what has been observed in cultured cells [7] . Presumably, the applied force on the embryo becomes distributed throughout the tissue changing the orientation of the maximum force vector on mitotic cells and the cells respond to reorient along the new axis. We went on to test if mechanical stimulation would lead to increased spindle rotation in FAK morphants. Despite the fact that under basal conditions FAK morphants display similar average spindle rotation and frequency of rotation with controls, under conditions of mechanical stimulation morphants fail to respond suggesting that FAK is required for the spindle rotation response ( Fig. 7a–c ). Owing to variations in the size of embryos that could lead to variations of the force exerted on each embryo, this experiment was repeated in embryos unilaterally injected with the FAK MO leading to similar results ( Supplementary Fig. 7a,b ). Decoupling the spindle from the cortex could explain this defect, however, high-resolution imaging of mitotic spindles of morphant cells revealed that both spindle capture and spindle centring are unaffected in agreement with the in vitro data showing that both spindle integrity and centring are unaffected in FAK-null cells ( Supplementary Fig. 7d ). Moreover, mitosis in FAK morphants progresses smoothly with no delays ( Supplementary Fig. 7c ). We went on to use laser ablation to generate pulling forces perpendicular to the axis of the spindle of mitotic cells in a similar approach to what was described by Campinho et al. [8] in Zebrafish. Two cells positioned above and below the mitotic cell in a line perpendicular to the orientation of the spindle were laser ablated. Laser ablation leads to the extrusion of the ablated cell creating a wound. As the epithelium stretches to close the wound, it imposes tension on the tissue between the ablation sites causing the mitotic cell to change shape and stretch along the axis perpendicular to the spindle. As shown, the spindle of the control cell begins to rotate concomitant with cell stretching eventually becoming aligned with the imposed force ( Fig. 8a,b ). In FAK morphants, however, the spindle fails to respond and remains at a right angle to the force vector ( Fig. 8a,b ). These results suggest that FAK is required for spindle reorientation in response to external forces. As mentioned above, the forces generated by the wounds deform the mitotic cell elongating it along the axis of force. Cells have been shown to orient their spindle in response to force and cell shape [6] , [7] , both of which share the same axis in the above experiment making the contribution of each parameter difficult to resolve. In an effort to pinpoint the defect, we carried out laser ablations of single cells at regions perpendicular to their long axis in high-salt conditions. Ablating a single cell ensured that wound-derived forces would not lead to large-cell shape changes and high salt that wounds would close rapidly giving rise to relatively brief application of force on the mitotic cell. Imaging of control cells in which a long axis was present before wound closure but the cell became symmetric after would closure revealed that the spindle rotates to align with the imposed force despite the absence of a clearly defined long axis ( Supplementary Fig. 8a ). Time-lapse imaging of cells under conditions where the original long axis remained after wound closure revealed that during wound closure, spindles display a transient rotation to align with the applied force but eventually realign (albeit not always completely) with the long axis, once the wound closes and presumably the applied force dissipates. These cells eventually divide along their long axis suggesting that spindle orientation is determined by a combination of both sensing of forces and cell shape ( Supplementary Fig. 8b ). The contribution of each parameter to the final spindle orientation is difficult to assess, however, the transient rotation in cells with a clearly defined long axis away from that axis suggests that external forces may override cell shape. We went on to carry out the same experiment in FAK morphant embryos, and in this case, cells failed to display any transient rotations as expected given their inability to rotate even in response to double wounds and significant cell shape change ( Supplementary Fig. 8c ). These data suggest that FAK is required in order for mitotic cells to respond to external forces and reposition their spindle but do not rule out the possibility that it is also required for orientation with respect to cell shape. If spindle orientation is determined via a multi-parameter mechanism where both external forces and cell shape contribute to the final axis of division, as the majority of cells would be elongated along the axis of greatest force, the synthesis of information would make alignment along the long axis more robust. It is possible that due to an inability to properly transduce force alignment cues, FAK morphants fail to align unless the cell shape anisotropy is very high. In order to address this possibility, we generated linear wounds on control and morphant tailbuds using the gastromaster microsurgery instrument. Embryos were allowed to heal and fixed an hour later, to allow for the tension within the tissue to subside. Cells from these embryos display a great range of shape anisotropy with cells close to the wounds becoming very elongated. Although imaging these cells it became evident that in FAK morphant cells that were highly anisotropic, the spindle was always oriented along the long axis just like in controls ( Fig. 8c,d ). Use of low-concentration nocodazole (Noc) to depolymerize astral microtubules in control embryos on the other hand, gave rise to mitotic cells which failed to become oriented along the long axis irrespective of the extent of cell shape anisotropy ( Fig. 8c,d ). Quantification of spindle angles in relation to shape anisotropy from control, FAK morphant- and Noc-treated embryos confirm these observations ( Fig. 8d ). Although FAK morphants fail to orient along the long axis at low cell shape anisotropy they start behaving like controls above a threshold (length to width ratio=3), whereas spindles of cells from Noc-treated embryos remain randomized irrespective of cell shape ( Fig. 8d ). Overall, the above data suggest that FAK is required for the transduction of mechanical signals from the cell exterior to the cortex, which in turn bias cortical cues resulting in correct spindle alignment. 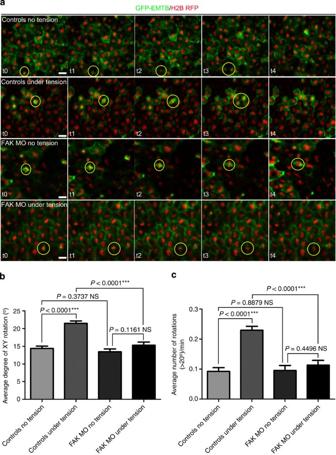Figure 7: FAK is required in the response of the spindle to external forces. (a) Stills (4 min interval) from time lapse recordings from stage 11 embryos expressing GFP-EMTB and histoneRFP, showing rotations of the mitotic spindle in controls and FAK morphant embryos under normal conditions and conditions of mechanical stimulation (MS). Yellow circles indicate representative mitotic cells from each condition. (b) The average spindle rotation for control embryos without MS is 14.41±0.6600° (n=267), for control embryos under MS is 21.51±0.6631° (n=405), for FAK morphants without MS is 13.48±0.7861° (n=165) and for FAK morphant embryos under MS is 15.33±0.8635° (n=174). Analysis of spindle rotation with a two-tailed unpairedt-test showed statistically significant differences of the means between controls without MS and controls under MS (***P<0.0001) and between controls under MS and FAK morphants under MS (***P<0.0001) but no statistically significant differences between controls without MS and FAK morphants without MS (not significant (NS):P=0.3737) or between FAK morphants without and with MS (NS:P=0.1161);n, number of spindle rotations, three independent experiments. Error bands are s.e.m. (c) Quantification of the frequency of mitotic spindle rotation. The average frequency of rotation per minute is 0.09238±0.01245 (n=82) for control embryos without MS, 0.2296±0.01329 (n=120) for control embryos under MS, 0.09532±0.01688 (n=47) for FAK morphants without MS and 0.1133±0.01588 (n=68) for FAK morphant embryos under MS. The results were analysed with a two-tailed unpairedt-test, showing statistically significant differences of the means of the rotation frequencies between controls without and with MS (***P<0.0001) and between controls under tension and FAK morphants under MS (***P<0.0001) but no statistically significant differences between controls and FAK morphants without MS (NS:P=0.8879) or between FAK morphants without and with MS (NS:P=0.4496);n, number of divisions. Scale bars (a), 20 μm. Figure 7: FAK is required in the response of the spindle to external forces. ( a ) Stills (4 min interval) from time lapse recordings from stage 11 embryos expressing GFP-EMTB and histoneRFP, showing rotations of the mitotic spindle in controls and FAK morphant embryos under normal conditions and conditions of mechanical stimulation (MS). Yellow circles indicate representative mitotic cells from each condition. ( b ) The average spindle rotation for control embryos without MS is 14.41±0.6600° ( n =267), for control embryos under MS is 21.51±0.6631° ( n =405), for FAK morphants without MS is 13.48±0.7861° ( n =165) and for FAK morphant embryos under MS is 15.33±0.8635° ( n =174). Analysis of spindle rotation with a two-tailed unpaired t -test showed statistically significant differences of the means between controls without MS and controls under MS (*** P <0.0001) and between controls under MS and FAK morphants under MS (*** P <0.0001) but no statistically significant differences between controls without MS and FAK morphants without MS (not significant (NS): P =0.3737) or between FAK morphants without and with MS (NS: P =0.1161); n , number of spindle rotations, three independent experiments. Error bands are s.e.m. ( c ) Quantification of the frequency of mitotic spindle rotation. The average frequency of rotation per minute is 0.09238±0.01245 ( n =82) for control embryos without MS, 0.2296±0.01329 ( n =120) for control embryos under MS, 0.09532±0.01688 ( n =47) for FAK morphants without MS and 0.1133±0.01588 ( n =68) for FAK morphant embryos under MS. The results were analysed with a two-tailed unpaired t -test, showing statistically significant differences of the means of the rotation frequencies between controls without and with MS (*** P <0.0001) and between controls under tension and FAK morphants under MS (*** P <0.0001) but no statistically significant differences between controls and FAK morphants without MS (NS: P =0.8879) or between FAK morphants without and with MS (NS: P =0.4496); n , number of divisions. Scale bars ( a ), 20 μm. 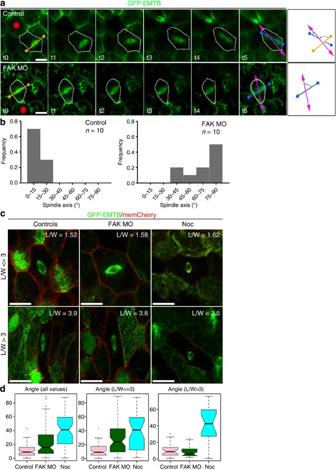Figure 8: FAK is required for the transduction of the extracellular forces to the cortex that guide spindle orientation. (a) Stills (2 min interval) from a time lapse recording where neighbouring cells of a mitotic cell were laser ablated (red star) to generate tension perpendicular to the initial axis of the spindle (orange axis). The white dashed line delineates the cell boundary. (b) Quantification was performed by measuring the angle (black dashed line) between the final spindle axis (blue) and the induced tension axis (magenta axis). The histograms show the frequency distributions of the observed angles for control and morphant embryos. A two-tailed unpairedt-test showed statistically significant differences of the means of the spindle angles between the two samples, ***P<0.0001; control spindle angle 10.99±2.417°, FAK MO spindle angle 67.04±5.671°, ten embryos per sample, two independent experiments. (c) Representative images of mitotic cells from wounded tailbuds that displayed small (L/W≤3) or large (L/W>3) shape anisotropy from control, FAK morphants and Noc-treated control embryos. (d) L/W ratio was calculated for each cell and correlated to the spindle angle, which was defined as the angle between the line connecting the two spindle poles and the long axis of the cell. Box-Whisker plots of the angle values are presented for the three experimental conditions. The first box-plot shows all the angles that were measured from all the cells from each sample, the second pox-plot shows angles measured from cells with L/W≤3 and the third box-plot angles measured from cells with L/W>3. Kruskal–Wallis test revealed that the three samples show statistical significant differences in each case (P<0.01). Mann–Whitney test between the three samples in the first box-plot showed that all three display statistically significant differences (P<0.01). In contrast, in the second plot (L/W≤3) only the comparisons between Control-FAK MO and Control-Noc display statistically significant differences (P<0.01), whereas FAK MO and Noc (P=0.22) do not. In the third box-plot (L/W>3) only the comparisons between Control-Noc and FAK MO-Noc display statistically significant differences (P<0.01), whereas control and FAK MO (P=1) do not. Scale bars (a,c,d), 20 μm. Full size image Figure 8: FAK is required for the transduction of the extracellular forces to the cortex that guide spindle orientation. ( a ) Stills (2 min interval) from a time lapse recording where neighbouring cells of a mitotic cell were laser ablated (red star) to generate tension perpendicular to the initial axis of the spindle (orange axis). The white dashed line delineates the cell boundary. ( b ) Quantification was performed by measuring the angle (black dashed line) between the final spindle axis (blue) and the induced tension axis (magenta axis). The histograms show the frequency distributions of the observed angles for control and morphant embryos. A two-tailed unpaired t -test showed statistically significant differences of the means of the spindle angles between the two samples, *** P <0.0001; control spindle angle 10.99±2.417°, FAK MO spindle angle 67.04±5.671°, ten embryos per sample, two independent experiments. ( c ) Representative images of mitotic cells from wounded tailbuds that displayed small (L/W≤3) or large (L/W>3) shape anisotropy from control, FAK morphants and Noc-treated control embryos. ( d ) L/W ratio was calculated for each cell and correlated to the spindle angle, which was defined as the angle between the line connecting the two spindle poles and the long axis of the cell. Box-Whisker plots of the angle values are presented for the three experimental conditions. The first box-plot shows all the angles that were measured from all the cells from each sample, the second pox-plot shows angles measured from cells with L/W≤3 and the third box-plot angles measured from cells with L/W>3. Kruskal–Wallis test revealed that the three samples show statistical significant differences in each case ( P <0.01). Mann–Whitney test between the three samples in the first box-plot showed that all three display statistically significant differences ( P <0.01). In contrast, in the second plot (L/W≤3) only the comparisons between Control-FAK MO and Control-Noc display statistically significant differences ( P <0.01), whereas FAK MO and Noc ( P =0.22) do not. In the third box-plot (L/W>3) only the comparisons between Control-Noc and FAK MO-Noc display statistically significant differences ( P <0.01), whereas control and FAK MO ( P =1) do not. Scale bars ( a , c , d ), 20 μm. Full size image FAK is required for epithelial morphogenesis In order to assess the significance of the spindle orientation defects arising from FAK loss of function in the embryo, we turned to two morphogenetic events known to require oriented cell divisions, epiboly and the development of the pronephros [43] , [48] . The Xenopus AC is initially three cell layers and rearranges into two layers via radial intercalation. This two-layer arrangement is maintained through oriented cell divisions at the plane of the epithelium [43] , [49] . We have previously shown that loss of FAK leads to block of epiboly through inhibition of radial intercalation and loss of spindle orientation [22] . In order to decouple the two processes and examine the effects of loss of spindle orientation on epithelial morphogenesis independently from radial intercalation, we generated an inducible FF dominant negative based on the hormone-binding domain of the glucocorticoid receptor [50] . The FF inducible construct was initially tested in adherent cells and as shown, in the absence of induction FF localizes primarily in the cytosol and becomes localized at FAs only upon induction ( Supplementary Fig. 9a ). We thus induced FF-injected embryos at stage 10.5 to ensure that radial intercalation had been completed and assessed blastopore closure and AC thickness. As shown, FF expression delayed blastopore closure ( Supplementary Fig. 9b ) and led to thickening of the AC ( Fig. 9a,b ), even after radial intercalation was completed, suggesting that loss of spindle orientation alone is sufficient to interfere with epiboly. In addition, the presence of heavily pigmented cells within the deep layers of the AC suggests that pigmented cells of the outermost epithelium divide asymmetrically, ingressing into the deep layer and contributing to the increase of AC thickness ( Fig. 9c,d ). These results show that FAK’s role in spindle orientation is indispensable for correct epithelial morphogenesis during epiboly [51] . 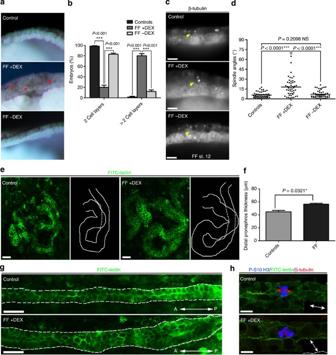Figure 9: FAK’s role in spindle orientation is important for epithelial morphogenesis. (a) Sectioned control, FF-injected and FF-injected and dexamethasone-treated (at stage 10.5) embryos. In FF+DEX embryos epiboly is blocked and pigmented cells of the outermost layer can be seen in the deep layers (red arrowheads). (b) Percentage of embryos with a two-cell layered AC at stage 12. 98.5% in controls (n=50), 20% in FF+DEX (n=71) and 83% in FF–DEX-injected embryos (n=26). Analysis with a two-way analysis of variance (ANOVA) test revealed that these differences are statistically significant (***P<0.001);n, number of embryos, two independent experiments. (c) Fluorescence images of mitotic spindles (yellow arrowheads) in sectioned control, FF-DEX and FF+DEX-injected embryos. (d) Scatter plots of the spindle angles. The average spindle angle in controls is 5.807±0.6240° (n=50), in FF+DEX is 18.05±1.924° (n=48) and in FF–DEX is 7.039±0.7434° (n=53). Quantification of spindle orientation with an unpairedt-test showed statistically significant differences of the mean spindle angle between controls and FF+DEX (***P<0.0001) and between FF+DEX and FF–DEX (***P<0.0001) but not between controls and FF–DEX-injected cells (not significant (NS):P=0.2098);n, number of metaphase cells, two independent experiments. (e) Maximum Intensity Projections fromZ-stacks of theXenopuspronephros including outlines of the distal pronephros from st.40 control and FF-injected embryos. (f) Quantification of distal pronephros thickness. The average diameter in controls is 44.52±0.8598 μm and in FF-injected is 56.33±1.396 μm. Analysis of the pronephros thickness with a two-way ANOVA test showed statistically significant differences of the means between the samples, *P<0.0321 (n=6;n, number of embryos). (g) Optical sections of the pronephric duct in control and FF-injected tadpoles. The white dashed line defines the pronephric duct. (h) Confocal images of mitotic spindles in the duct of control and FF-injected tadpoles. In control cells, the mitotic spindle is parallel to the long axis of the duct, whereas in FF-injected cells, it is oriented orthogonally to the long axis of the duct. The black boxes show a schematic diagram of how the spindle is oriented (white axis) with respect to the duct lumen (dashed line). Scale bars (c), 20 μm, (e,g) 50 μm, (h) 10 μm. Figure 9: FAK’s role in spindle orientation is important for epithelial morphogenesis. ( a ) Sectioned control, FF-injected and FF-injected and dexamethasone-treated (at stage 10.5) embryos. In FF+DEX embryos epiboly is blocked and pigmented cells of the outermost layer can be seen in the deep layers (red arrowheads). ( b ) Percentage of embryos with a two-cell layered AC at stage 12. 98.5% in controls ( n =50), 20% in FF+DEX ( n =71) and 83% in FF–DEX-injected embryos ( n =26). Analysis with a two-way analysis of variance (ANOVA) test revealed that these differences are statistically significant (*** P <0.001); n , number of embryos, two independent experiments. ( c ) Fluorescence images of mitotic spindles (yellow arrowheads) in sectioned control, FF-DEX and FF+DEX-injected embryos. ( d ) Scatter plots of the spindle angles. The average spindle angle in controls is 5.807±0.6240° ( n =50), in FF+DEX is 18.05±1.924° ( n =48) and in FF–DEX is 7.039±0.7434° ( n =53). Quantification of spindle orientation with an unpaired t -test showed statistically significant differences of the mean spindle angle between controls and FF+DEX (*** P <0.0001) and between FF+DEX and FF–DEX (*** P <0.0001) but not between controls and FF–DEX-injected cells (not significant (NS): P =0.2098); n , number of metaphase cells, two independent experiments. ( e ) Maximum Intensity Projections from Z -stacks of the Xenopus pronephros including outlines of the distal pronephros from st.40 control and FF-injected embryos. ( f ) Quantification of distal pronephros thickness. The average diameter in controls is 44.52±0.8598 μm and in FF-injected is 56.33±1.396 μm. Analysis of the pronephros thickness with a two-way ANOVA test showed statistically significant differences of the means between the samples, * P <0.0321 ( n =6; n , number of embryos). ( g ) Optical sections of the pronephric duct in control and FF-injected tadpoles. The white dashed line defines the pronephric duct. ( h ) Confocal images of mitotic spindles in the duct of control and FF-injected tadpoles. In control cells, the mitotic spindle is parallel to the long axis of the duct, whereas in FF-injected cells, it is oriented orthogonally to the long axis of the duct. The black boxes show a schematic diagram of how the spindle is oriented (white axis) with respect to the duct lumen (dashed line). Scale bars ( c ), 20 μm, ( e , g ) 50 μm, ( h ) 10 μm. Full size image Another tissue in which oriented cell divisions are known to be important is the kidney. A model has emerged in which oriented cell divisions are critical for the normally thin elongated tubes to develop, with evidence suggesting that misoriented divisions lead to cystic kidney disease in animal models [52] . We thus targeted the inducible FF at the pronephros and induced the construct at stage 32/33. FF expression resulted in spindle misorientation and pronephros defects including dilated tubules, whereas the pronephric duct was also dilated compared with that of controls ( Fig. 9e–h ). Overall, these data suggest that FAK’s role in spindle orientation is important for epithelial morphogenesis. In this manuscript, we provide evidence for the involvement of FAK in spindle orientation both in cultured cells as well as in the epithelia of the developing vertebrate embryo. We provide evidence that spindle integrity, centring and cortical microtubule capture are unaffected in the absence of FAK, yet these cells fail to respond to external forces suggesting that FAK’s involvement in spindle orientation stems from a defect in the transmission of external forces to the cell cortex. Furthermore, our results suggest that an interaction between FAK and paxillin is critical for FAK’s role in spindle positioning, whereas FAK’s kinase activity is dispensable in this context, revealing the first kinase domain dependent but kinase activity independent function of FAK. Although the requirement for the presence of the kinase domain suggests a scaffolding function for this domain, it is also possible that its presence is required in order to regulate or stabilize the conformation of the adjacent proline-rich regions or even that basal kinase activity is retained in the K454R mutant and is sufficient for this particular function. FAK-null cells display RFs during mitosis in a similar manner as FAK reconstituted cells, yet fail to orient their spindle parallel to the matrix, whereas they also fail to orient according to extracellular cues in the XY plane. These results suggest that the presence of RFs is not sufficient for force transmission to the cortex of adherent cells but rather that forces are transmitted via a cytoskeletal link to the adhesive complex itself. Our results suggest that despite the fact that the majority of FAs disassemble during mitosis, a FAK-positive basal FA complex is retained at the RF–ECM interface. The composition of this complex warrants further study to determine which FA proteins other than FAK and paxillin remain localized at RFs during mitosis. We propose that these retraction adhesions anchor actin filaments to the ECM and through these, forces are transmitted to the cell cortex. In the early embryo, the situation is different. The cells of the prospective neurectoderm encompass the entire embryo during gastrulation via epiboly, and at the end of gastrulation, the epithelium is composed of two cell layers [49] . The outer cells are attached to one another via tight junctions at their apical surface and via adherens junctions in their lateral regions [53] , [54] . They are also anchored to the deep cell layer via adherens junctions and only the deep layer is in contact with the ECM [55] . This suggests that cell–ECM interactions are not important for spindle orientation in the outer epithelium. This is also supported by the fact that fibronectin MOs as well as fibronectin antibodies that disrupt the fibronectin matrix assembly, thus disrupting cell–ECM interactions, fail to affect oriented cell divisions in the outer epithelial layer [43] , [56] . If cell–ECM interactions are dispensable for oriented divisions in the outer epithelium, is then FAK’s role in this context integrin independent? As cadherins have been shown to be required for proper spindle orientation, it is possible that FAK acts through adherens junctions to position the spindle in the epithelium, especially given the fact that both FAK and paxillin have been shown to influence adherens junctions or interact with adherens junction proteins [57] , [58] . In addition, as we show, both FAK and paxillin co-localize with the adherens junctions of epithelial cells and are enriched at the apical region of the cell cortex in the outer epithelium of Xenopus . Another interesting possibility is that the role of integrins in epithelial tissue spindle orientation is independent from their role in cell–ECM interactions and FAK’s role in this context is again stemming from the transduction of integrin-dependent signals. Support for this notion comes from studies in the fly showing that although integrin signalling is required for the correct orientation of the mitotic apparatus and maintenance of the ovarian monolayer epithelium, cell–ECM interactions are dispensable [59] . Although significant progress has been made towards understanding how cells couple cortical polarity signals and spindle positioning, how cells receive external stimuli and how these are translated at the cortex are poorly understood [3] . During early embryonic development, mechanical forces are believed to play a critical role in morphogenesis in part through control of cell division orientation [60] . Experiments in zebrafish showed that tissue level forces orient the mitotic spindle during epiboly thus releasing anisotropic tension in the EVL [8] . We show that in a similar manner, external forces can orient mitotic cells in Xenopus epithelia and provide direct evidence that FAK is required for spindle responses to such forces. Although both force and cell shape have been shown to control spindle orientation, our results suggest that the primary defect of FAK downregulation is loss of the ability to orient depending on force, given the fact that in the presence of high cell shape anisotropy, FAK morphants orient correctly. FAK, however, is not only required for epithelial cells to orient their spindle along force vectors but it is also required to maintain cell divisions in the plane of the epithelium. This is in agreement with data in Medaka showing that planar divisions in the neuroepithelium are randomized in FAK morphant cells [61] . We show that blocking FAK function after radial intercalation has been completed, leads to failure of epiboly suggesting that correct spindle orientation is necessary for epithelial spreading, an important morphogenetic process shared by all vertebrates [51] . Blocking FAK function also leads to defective pronephros development highlighting the importance of proper spindle orientation in organogenesis. Overall, our work identifies a novel role for FAK in spindle orientation and consequently for epithelial morphogenesis and reveals that this role stems from FAK’s role in the transduction of external orienting forces to the cell cortex. We have recently shown that FAK is also involved in motile ciliogenesis by regulating ciliary adhesions, complexes formed at the basal bodies linking them to the actin cytoskeleton [40] . Thus, FAK is joining a number of proteins involved in both spindle orientation and cilia formation like IFT88, Msd1/SSX2IP Wtip and Vangl2 (refs 62 , 63 , 64 ). At least in one case, that of IFT88, it has been shown that the role in spindle orientation is not secondary to the protein’s role in ciliogenesis, but independent [65] . Similarly, in the case of FAK, we propose that the two roles are distinct and stem from FAK’s regulation of related but different complexes. Cell culture The FAK−/− cell line (American Type Culture Collection (ATCC)) was cultured in DMEM with 10% fetal bovine serum (FBS) and 1 mM sodium pyruvate at 37 °C. HeLa (ATCC) and NIH3T3 (ATCC) cells were cultured in DMEM with 10% FBS at 37 °C. All cell lines were transfected with the indicated plasmids using Lipofectamin 2000 (11668019, Invitrogen) according to the manufacturer’s protocol. FAK inhibitor PF-228 (Sigma) was added in HeLa and NIH3T3 cells at 10 and 5 μM for 24 h, respectively. Dexamethasone was added in HeLa cells at a concentration of 100 nM for 3 h. XL177 cells [66] were cultured in 70% L-15, 15% FBS and 100 mM L -glutamine at room temperature (RT), XL177 cells were transfected by electroporation (Invitrogen). Plating of the FAK −/− cells on fibronectin micropatterned coverslips (CYTOO) was performed according to the manufacturer’s protocol. Three-dimensional adhesion assay The adhesion of HeLa cells between two coverslips was performed as follows: Bottom coverslips were charged, spotted with silicone grease at the edges and then coated with 50 μg ml −1 fibronectin (33010-018, Invitrogen) for 1 h at 37 °C. Top coverslips were also charged and coated either with poly- L -lysine (P8920, Sigma) or fibronectin. Cells were seeded on the bottom fibronectin-coated coverslips and allowed to adhere for 15 min. After initial attachment and while cells were still round, the second coverslip was secured in place on top using the silicone grease spots and carefully lowered under an inverted microscope until it contacted the cells. Cells were grown for 6 h at 37 °C and then were either imaged live or fixed and processed for immunofluorescence. DNA constructs and MO oligonucleotides All plasmids generated were verified by sequencing. The green fluorescent protein (GFP) and haemagglutinin (HA)-tagged versions of FAK, FRNK and FF plasmids have been described [22] , [44] . The HA FAK-K454R pCS2 ++ construct was generated by subcloning from the pKH3 HA FAK-K454R plasmid (kindly provided by the Guan lab) using the primers F/HA: 5′-ATGCGGCCGCATGTACCCATACGATGTTCCAGATTCCGCT-3′ and R/FAK: 5′-TTTCTCGAGTTAGTGGGGCCTGGACTGGCTGATCATTTT-3′. The GFP FAKΔFAT pCS108 construct was generated by PCR using the primers F/GFP: 5′-AAAGCGGCCGCATGGTGAGCAAGGGCGAGGAGCTG-3′ and R/ΔFAT: 5′-AACTCGAGTCTTCACGCCTTCGTTGTAGCTGTCCACGGGG-3′ and the template of GFP FAK pCS2 ++ . The HA ΔFERM/K454R pCS2 ++ construct was generated by subcloning a fragment of FAK containing the K454R mutation form the HA FAK-K454R pCS2 ++ plasmid followed by ligation to the plasmid of HA ΔFERM pCS2 ++ (ref. 44 ). The plasmids HA FAK-L1034S, GFP FAK-L1034S and GFP FAK-E1015A were generated by site-directed mutagenesis using the set of primers F/FAK-L1034S: 5′-GCTGTGGATGCCAAGAACTCGCTGGATGTCATCGATCAAGC-3′, R/FAK-L1034S: 5′-GCTTGATCGATCACATCCAGCGAGTTCTTGGCATCCACAGC-3′ for the L1034S mutation and the set of primers F/FAK-E1015A: 5′-CCAGCCTGCAGCAGGCGTACAAGAAGCAAATGCT-3′ and R/FAK-E1015A: 5′-AGCATTTGCTTCTTGTACGCCTGCTGCAGGCTGG-3′ for the E1015A mutation. The GFP paxillin Rescue pCS2 ++ construct was generated by a two-step directed mutagenesis, mutating the sequence recognized by Paxillin MO using the primers F/Pxn Rescue 1: 5′-ATGGAAGAATTCGACGCCCTGCTGGCGGACTTGGAGTCTACC-3′ and R/Pxn Rescue 1: 5′-GGTAGACTCCAAGTCCGCCAGCAGGGCGTCGAATTCTTCCAT-3′ for the first step and the primers F/Pxn Rescue 2: 5′-ATGGAAGAATTCGATGCGCTCTTGGCGGACTTGGAGTCTACC-3′ and R/Pxn Rescue 2: 5′-GGTAGACTCCAAGTCCGCCAAGAGCGCATCGAATTCTTCCAT-3′ for the second step. The inducible FF dominant negative was generated in a three-step cloning as described below. Initially, a GFP-fused form of the FERM domain was amplified from the GFP FAK pCS2 ++ plasmid and cloned into the pCS108 vector using the primers F/GFP2: 5′-AAAGGATCCATGGTGAGCAAGGGCGAGGAGCTG-3′ and R/FERM: 5′-TTTGCGGCCGCATCTATTATCTCTGCATAGTCATCTGT-3′. Then the hormone-binding domain of the glucocorticoid receptor was PCR out from the Xbra-GR pSP64T plasmid (provided from Masazumi Tada lab) using the primers F/GR: 5′-AAAGCGGCCGCATCTGAAAATCCTGGTAACAAAACA-3′ and R/GR: 5′-TTTGATATCCTTTTGATGAAACAGAAGTTT-3′ and ligated to the GFP-FERM part in pCS108. Finally, the C-terminus FRNK domain was amplified from the GFP FAK pCS2 ++ plasmid and cloned into the GFP-FERM-GR part by using the primers F/FRNK_linker: 5′-AAGATATCGGTAGCGGCAGCGGTAGCAGGTTTACTGAACTTAAAGCAC-3′ and R/FAK, generating in this way an inducible from of the FF dominant negative with a GFP-tag on the N-terminus and the hormone-binding domain of the GR receptor in the middle of the construct. The plasmids membraneCherry pCS2 + and histoneGFP pCS2 + were kindly provided by Chenbei Chang lab. The HA-Par6 pCS2+ plasmid was provided from Ira O. Daar lab. The H2B-mRFP1 pCS2 plasmid was provided by Reinhard Koster lab. The EMTB-3xGFP pCS2 was provided by Brian J. Mitchell lab. The pEGFP C1-LGN construct was kindly provided by Fumiko Toyoshima Lab. All FAK mutants were generated from the FAK chicken variant (GenBank AAA48765.1). The sequence of FAK MO is 5′-TTGGGTCCAGGTAAGCCGCAGCCAT-3′ (ref. 21 ) and of Paxillin MO is 5′-CAGCAATGCATCCAGGTCATCCATG-3′. This MO is based on a previously published Paxillin MO with slight differences [47] . Embryos and manipulations Xenopus laevis embryos were staged according to the study by Nieuwkoop and Faber (1967). Embryos were fertilized in vitro and dejellied using 1.8% L -cysteine, pH 7.8, then maintained in 0.1 × Marc’s Modified Ringer’s (0.1xMMR). Microinjections were performed in 4% Ficoll in 0.3xMMR. Microinjections for the targeting of the AC performed at the one-cell stage, whereas microinjections for the targeting of the pronephros were performed at the two ventral vegetal blastomeres of eight-cell stage embryos. ACs were dissected from stage 9 embryos and cultured in DFA (53 mM NaCl 2 , 5 mM Na 2 CO 3 , 4.5 mM potassium gluconate, 32 mM sodium gluconate, 1 mM CaCl 2 , 1 mM MgSO 4 ) until stage 15, when they were fixed and processed for immunofluorescence. In order to generate high shape anisotropies in outer epithelial cells, linear parallel wounds were generated along the anterior–posterior axis of the embryo using the gastromaster microsurgery instrument. Embryos were allowed to heal in 1/3XMMR and were then fixed and imaged. Noc was used at 50 nM and was added to the embryos 20 min after the wounds were made and left for 40 min until fixation. Activation of the inducible FF dominant negative for the radial intercalation experiments was performed by incubation of stage 10.5 embryos in 10 μM dexamethasome (sc-29059, Santa Cruz) at 14 °C. Activation of the inducible FF for the evaluation of the effects on pronephros morphogenesis was performed by incubating the embryos with 10 μM dexamethasome in 0.1xMMR from stage 33/34 until either stage 35/36 for imaging cell divisions or stage 40 for evaluation of the pronephros morphology. Imaging Embryos were imaged either under a Zeiss Axio Imager Z1 microscope, using a Zeiss Axiocam MR3 and the Axiovision software 4.8, or a Zeiss LumarV12 stereomicroscope or under a laser scanning confocal LSM710 microscope (Zeiss). Live imaging of cell divisions described in Fig. 7 was performed as mentioned below. Imaging of gastrula embryos under conditions of reduced tension was performed by placing the embryos on a drop of Vaseline in a slide with a 2-mm silicone gasket and held in place by a glass coverslip, which was not in contact with the embryo. Optical sections were acquired every 2 min for a 40-min period. Imaging of embryos under conditions of increased tension was performed by placing the embryos in a slide with a 1-mm silicone gasket, applying in this way external mechanical force directly on the embryo and imaged as described above. Laser ablation experiments were conducted using the LSM 710 confocal microscope and a Plan-Apochromat × 63/1.40 Oil DIC M27 objective lens (Zeiss). An early mitotic cell was selected and an image was acquired to determine the orientation of the division axis. For the data presented in Fig. 7a , wounds were performed in the two neighbouring cells in the axis perpendicular to the long axis of the spindle by using the 488- and 543-nm laser lines simultaneously, 50 iterations at 100% power and the mitotic cell was imaged every 15 s until the beginning of cytokinesis. For the data presented in Supplementary Fig. 7c,d,e, laser ablations were contacted as described above with the differences that the embryos were placed in high-salt solution (1x3 MMR) and only one cell near the mitotic cell was ablated in order to create a smaller wound that will not cause severe cell deformation. Image of the spindle capture to the cell cortex was performed by using the LSM 710 confocal microscope and a Plan-Apochromat × 63/1.40 Oil DIC M27 objective lens (Zeiss) in embryos expressing GFP-EMTB and memCherry. Immunofluorescence Immunofluorescence on FAK−/−, HeLa, XL177 and NIH3T3 cells was carried out as follows: cells were plated on glass coverslips washed three times with PBS and then fixed for 10 min in 4% paraformaldehyde solution. Fixation was followed by addition of 50 mM glycine solution and then the cells were permeabilized using 0.2% Triton-X solution for 10 min. Permeabilized cells were blocked using 10% normal donkey or goat serum (017-000-121, Jackson Immunoresearch or 16210072, Invitrogen) for 30 min. Cells were incubated with primary antibodies for 1 h. Primary antibodies used were: β-tubulin (1:200, E7-c, Hybridoma Bank), Histone H3 phosphorylated Ser10 (1:1,000, 06-570, Millipore), HA (1:500, sc-805, Santa Cruz) and Paxillin (1:750, 610569, BD Biosciences). Cells were then washed several times in PBS. Secondary antibodies used were Cy3 (1:500, 711-165-152 or 715-165-150, Jackson Immunoresearch), Alexa fluor 488 (1:500, A11029 or A11034, Invitrogen), Alexa fluor 633 (1:500, A21052 or A21070, Invitrogen). Phalloidin was incubated together with the secondary antibodies, phalloidin 488 (1:500, A12379, Invitrogen), phalloidin 633 (1:500, A22284, Invitrogen). Immunfluorescence of Xenopus ACs was performed as whole mount immunostaining. ACs were fixed in 10% 10XMEMFA (0.1 mM 3-( N -morpholino)propanesulfonic acid, pH 7.4, 2 mM EGTA, 1 mM MgSO 4 ), 3.7% formaldehyde–10% formaldehyde and 80% water for 2 h at RT, dehydrated in ethanol and permeabilized for 2 h in 1 × PBS, 0.5% Triton, 1% dimethyl sulfoxide and blocked for 1 h in 10% Normal Goat or Normal Donkey serum. Primary antibodies used were: GFP (1:500, A11122, Invitrogen), HA (1:250, sc-805, Santa Cruz), β-tubulin (1:200, E7-c, Hybridoma Bank), ZO-1 (1:500, 61-7300, Invitrogen), Histone H3 phosphorylated Ser10 (1:1,000, 06-570, Millipore), aPKC (1:250, sc-216, Santa Cruz), FAK (1:100, 05-537, Millipore), Paxillin (1:500, 610569, BD Biosciences), β-catenin (1:500, sc-7199, Santa Cruz). The incubation was performed overnight at 4 °C. ACs were then washed four times for 20 min, incubated for 2 h RT with secondary antibodies: Alexa fluor 488 (1:500, A11029 or A11034, Invitrogen), Cy3 (1:500, 715-165-150 or 711-165-152, Jackson Immunoresearch) Alexa fluor 633 (1:500, A21052 or A21070, Invitrogen), at RT and then washed several times and post-fixed in 1XMEMFA. Clearing of the ACs was performed by immersing the embryos in Murray’s Clearing Medium. Immonofluorescence for the Xenopus pronephros was performed as whole-mount immunostaining with the difference that the tadpoles were treated with 0.01% Triton in 0.1xMMR prior fixation to avoid staining of the epidermis in order to facilitate imaging of the deep tissue. FITC-labelled Lycopersicon Esculentum (Tomato) Lectin (1:500, FL-1171, Vector Labs) was used for pronephros staining together with the secondary antibodies. Western blot Protein lysates were prepared by homogenizing cells or embryos in ice-cold radioimmunoprecipitation assay lysis buffer (50 mM Tris–HCl, pH 7.4, 150 mM NaCl, 2 mM EDTA, 1% NP-40, 0.1% SDS, 1% deoxycholate 24 mM) supplemented with phosphatase inhibitors (5 mM sodium orthovanadate, Na 3 VO 4 ) and protease inhibitors (1 mM phenylmethanesulfonyl fluoride, Protease cocktail, Sigma). Homogenates were cleared by centrifugation at 10,000 g for 5 min at 4 °C for cells or at 15,000 g for 30 min at 4 °C for embryos. Protein levels were determined by bicinchoninic acid assay using the Magellan Data Analysis software (Tecan). The lysates were loaded on 7.5% SDS–polyacrylamide gels with the WesternC ladder (161-0376, Bio-Rad). The proteins were transferred onto nitrocellulose membrane, blocked in 5% milk (in TBST: 1 × TBS and 0.1% Tween). The blotting was performed by incubation of the primary antibodies overnight at 4 °C. Blots were incubated with N-FAK mouse monoconal (1:500, 05-537, Millipore), P-Y397 rabbit polyclonal (1:1,000, ab4803, Abcam), P-Y576 recombinant monoclonal (1:500, 700013, Invitrogen), Paxillin (1:5,000, 610569, BD Biosciences) and actin (1:1,000, sc-1616, Santa Cruz). Visualization was performed using HRP-conjugated antibodies (1:15,000, sc-2301 or sc-2302, Santa Cruz) and detected with LumiSensor (GeneScript) on UVP iBox. Statistical analysis Quantification of the orientation of the division axis of metaphase cultured and epithelial cells were carried out with the ImageJ software by using the Z-projections of the images, where the angle between the line from the one spindle pole parallel to the substrate and the line connecting the two spindle poles was measured. Statistical analysis including analysis of variance and two-tailed unpaired t -test for parametric distributions and Kruskal–Wallis and Mann–Whitney tests for non-parametric distributions and graph construction was performed by the GraphPad software. The spindle size was determined by measuring the length and width of the mitotic spindle of metaphase cells. Maximum intensity projections were used for the measurements. The width was measured at the widest point of the mitotic spindle, usually at the centre of the spindle. As in the three dimensions, the spindle angle must also be considered and the actual length corresponds to the hypotenuse of the right triangle that connects the two poles, we calculated the length of the mitotic spindle as cos α / A , where α is the average spindle angle and A the length of the spindle in the maximum intensity projections. This process was performed both in control and experimental samples. Spindle centring was calculated by measuring the distance from each spindle pole of a metaphase cell to the nearest point at the cell cortex and then the distance with the greatest value was divided by the distance with the smallest value. Off centre spindles were defined when the above ratio was greater than 1.5. The correlation of the spindle poles to the LGN cortical crescent was performed by measuring the angle formed between the line connecting the centre of the metaphase plate perpendicularly to the cell cortex and the line extending from the centre of the LGN cortical crescent towards the centre of the metaphase plate. The spindles that displayed an angle between 30° and 90° were considered as uncoupled with the LGN cortical localization. The average degree of spindle rotation in Xenopus embryos was calculated by ImageJ and Graphpad software, where the angle between the long axis of the spindle at the first time and the next time point was measured. In order to calculate the average number of spindle rotations per frame, for each metaphase cell, the number of rotations above 20° was counted and divided by the number of total rotations. The frequency was calculated by dividing this result with the time interval between the frames. The quantification of the spindle rotation after laser ablation was performed by measuring the angle between the final division axis before cytokinesis and the axis of the induced tension which corresponds to the long axis of the cell after it changes its shape. Histograms were generated with the GraphPad software where the frequency of the above spindle angle was calculated as the number of divisions that had a spindle angle in the indicated categories divided by the total number of divisions. The correlation between cell shape and spindle angles was determined by measuring the length and width for each cell as well as the angle of deviation of each spindle from the cells long axis. For the statistical analysis both Kruskal–Wallis and Mann–Whitney tests were performed between controls, FAK MO- and Noc-treated cells comparing all values or after setting a length to width ratio (L/W) threshold of three. The average thickness of the Xenopus distal pronephros was quantified by measuring the thickness of the pronephros in 20 different areas of the distal part in each embryo by using the Zen2009 Light Edition Software. The average thickness in each embryo was used for the two-way analysis of variance test to compare the thickness in control and experimental samples by using the GraphPad software. How to cite this article: Petridou, N. I. & Skourides, P. A. FAK transduces extracellular forces that orient the mitotic spindle and control tissue morphogenesis. Nat. Commun. 5:5240 doi: 10.1038/ncomms6240 (2014).